Mechanisms underlying beneficial plant–fungus interactions in mycorrhizal symbiosis Owing to their filamentous organization, fungi exploit very diverse substrates on the basis of their nutritional strategy. Saprobes thrive in soil, water and on decaying animal and plant tissues. A smaller group of fungi, the parasitic and mutualistic symbionts, feed on living organisms [1] . Such a classification cannot easily be applied to mycorrhizal fungi, a heterogeneous group of species spread over diverse fungal taxa. Although they can spend part of their life cycle as free-living organisms, mycorrhizal fungi always associate with the roots of higher plants, indeed over 90% of plant species, including forest trees, wild grasses and many crops. Both partners benefit from the relationship: mycorrhizal fungi improve the nutrient status of their host plants, influencing mineral nutrition, water absorption, growth and disease resistance, whereas in exchange, the host plant is necessary for fungal growth and reproduction [2] . Mycorrhizal fungi colonize environments such as alpine and boreal zones, tropical forests, grasslands and croplands. They have a major role in nutrient cycling through the specific activity of their mycelium in absorbing soil nutrients and supplying them to the plant, although their role in carbon flux is less well defined [3] . The term mycorrhiza is derived from the Greek words for 'fungus' and 'root'. Mycorrhizal fungi develop an extensive hyphal network in the soil, the aptly named wood-wide web [4] , which can connect whole plant communities offering efficient horizontal transfer of nutrients. Mycorrhizas develop specialized areas, called symbiotic interfaces, to interact with the host plant [5] , [6] , [7] . Mycorrhizal fungi can be divided into two major groups: aseptate endophytes such as Glomeromycota, or septate Asco- and Basidiomycota (see Box 1 Glossary) [2] . More commonly, mycorrhiza classifications reflect anatomical aspects and identify two broad categories [2] , referred to as ectomycorrhizas (EMs) and endomycorrhizas, depending on whether the fungus colonizes the root intercellular spaces or develops inside cells ( Fig. 1 ). Endomycorrhizas are further divided into orchid, ericoid and arbuscular mycorrhizas (AMs). 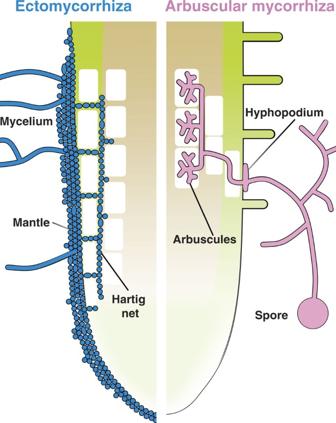Figure 1: Illustration of root colonization structures in ectomycorrhizal (blue) and arbuscular mycorrhizal (pink) interactions. The ectomycorrhizal fungus surrounds the root tip with a thick mantle of closely appressed hyphae, whereas the Hartig net develops around epidermal cells (green). In the case of arbuscular mycorrhizas, the root tip is usually not colonized. Hyphae develop from a spore and produce a hyphopodium on the root epidermis. Intraradical colonization proceeds both intra and intercellularly and culminates with the formation of arbuscules, little fungal trees, inside inner cortical cells (brown). Figure 1: Illustration of root colonization structures in ectomycorrhizal (blue) and arbuscular mycorrhizal (pink) interactions. The ectomycorrhizal fungus surrounds the root tip with a thick mantle of closely appressed hyphae, whereas the Hartig net develops around epidermal cells (green). In the case of arbuscular mycorrhizas, the root tip is usually not colonized. Hyphae develop from a spore and produce a hyphopodium on the root epidermis. Intraradical colonization proceeds both intra and intercellularly and culminates with the formation of arbuscules, little fungal trees, inside inner cortical cells (brown). Full size image A descriptive approach has dominated the investigation of mycorrhizas for at least 50 years until the advent of molecular biology, and the 'omics' era provided insight into their mechanisms. High-throughput technology, genome sequencing of fungi, plants and associated microbes, transcriptomic analyses, availability of mutant collections, RNA interference lines and plants transformed with fluorescent tags have all led to new perspectives on plant–microbe interactions, and on EMs and AMs in particular. In this review we focus on the mechanisms that govern the growth of EM and AM fungi and their interactions with plants. We report how genomics have unwrapped the genomes of at least two EM fungi, revealing their peculiarities, whereas similar approaches have not fully deciphered any AM fungal genome so far. By contrast, recent discoveries have shed light on the plant mechanisms that regulate AM interactions, mostly because of plant-based genetics, 'omics' and advanced microscopy technologies. Box 1: Glossary Trees in the families Pinaceae, Fagaceae, Dipterocarpaceae and Caesalpinoidaceae found in many forests all interact with hundreds of EM species of Basidiomycetes and Ascomycetes, so that these fungi can be said to have shaped the present forests [2] . EM fungi colonize the lateral roots of these trees with sheathing mycorrhizas, in which a fungal mantle covers the root tip, and a so-called Hartig net of intercellular hyphae surround epidermal and outer cortical cells ( Figs 1 and 2 ). EM fungi may also live independently of plant roots, as demonstrated by their growth capabilities in Petri dishes [2] . 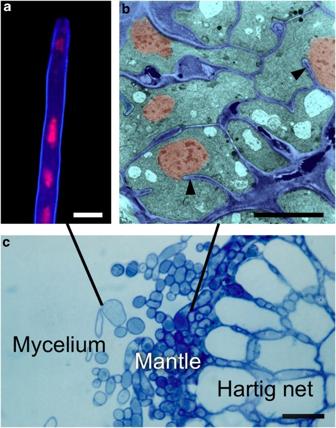Figure 2: The transition from the free-living status of an EM fungus to the symbiotic phase. A growing hypha from the mycelium ofT. melanosporumas observed in fluorescence microscopy is shown ina(courtesy: R. Balestrini). Hyphal morphology changes in the mantle, in which the repeated branching, characterized by incomplete transversal walls (arrowheads), originates a pseudoparenchymatous structure, as evident in the electron micrograph shown inb. In both images, the fungal wall is falsely coloured in blue and nuclei in red. The transverse section of a mycorrhizal root tip stained with Trypan blue is presented inc, showing the organization of hyphae in the mycelium, mantle and Hartig net. Bars, 10 μm. Figure 2: The transition from the free-living status of an EM fungus to the symbiotic phase. A growing hypha from the mycelium of T. melanosporum as observed in fluorescence microscopy is shown in a (courtesy: R. Balestrini). Hyphal morphology changes in the mantle, in which the repeated branching, characterized by incomplete transversal walls (arrowheads), originates a pseudoparenchymatous structure, as evident in the electron micrograph shown in b . In both images, the fungal wall is falsely coloured in blue and nuclei in red. The transverse section of a mycorrhizal root tip stained with Trypan blue is presented in c , showing the organization of hyphae in the mycelium, mantle and Hartig net. Bars, 10 μm. Full size image Molecular techniques have identified EM fungi in the field [8] , and owing to metagenomics, that is, the deep sequencing of organisms living in an environment [9] , a multitude of sequences from soil [10] are catalogued, also highlighting the rhizosphere around EMs as a special biome. Use of the Roche 454 Titanium genome sequencer has revealed unexpected levels of fungal biodiversity when applied to the soil of a French forest, in which Agaricomycetes were found to be the dominant class including a large number of EM species [11] . These data confirm that EM fungi have a dual lifestyle: they live as symbionts with plant roots and as facultative saprotrophs in soil [12] . However, data on their in situ activity (metatranscriptomics) are not yet available and the ecological functions accomplished by EM fungi in the soil remain at the moment unexplored. Genome sequencing of two EM fungi, the Basidiomycete Laccaria bicolor [13] and the Ascomycete Tuber melanosporum (black truffle) [14] , has shed some light on EM biology, highlighting similarities and differences between the two fungal symbionts and identifying the primary factors that regulate mycorrhiza development and function. Although L. bicolor has a 65-Mb genome and an estimated 19,102 protein-encoding genes, T. melanosporum , with its 125-Mb genome and an estimated 7500 protein-encoding genes, is in the odd condition of being the largest sequenced fungal genome, with a relatively small expected proteome compared with other filamentous fungi [14] . This argues that the symbiotic status can be achieved even with a reduced number of protein-coding genes, very few of which (1.5%) are differentially regulated during mycorrhizal formation [14] . Another contrasting feature is that the genome of L. bicolor has undergone extensive expansion of a few gene families with predicted roles in protein–protein interactions and signal-transduction mechanisms [13] , whereas this trait has not been observed in T. melanosporum , in which multigene families are rare. The genome size of both EM fungi is not ascribed to large-scale duplication events, but rather to a high number of transposable elements that represent more than 20 and 58% of the genome in L. bicolor [13] and T. melanosporum [14] , respectively. In the truffle, the insertion of transposable elements has been dated to 2–5 million years ago, and is considered to have contributed to genome evolution and plasticity. In filamentous Ascomycetes and Basidiomycetes, sexual fertilization and karyogamy are limited by a system of mating types, whereby only different and compatible strains can mate. T. melanosporum possesses the sex-related components identified in other Ascomycetes [14] , and the presence of HGM and MATa loci in the sequenced strain and in environmental samples shows that truffle is an obligate outcrossing species [15] . This is leading to the development of new strategies for truffle cultivation. Comparison of L. bicolor and truffle genomes with those of saprotrophic and pathogenic fungi reveals some components of the gene set required for a symbiotic lifestyle [12] . Both EM fungi have a relatively small number of enzymes that target plant cell wall components, for example, pectinases and pectin lyases. Remarkably, genes encoding some of these enzymes are upregulated during the symbiotic steps, when the fungus develops inside plant tissues. These data strongly suggest that the colonization process is based on limitation of host damage, avoiding the stimulation of defence reactions. The enzyme repertoire of both EM fungi also sheds light on their saprotrophic capacities. L. bicolor possesses substrate-degrading enzymes, including glycosyl hydrolases involved in the hydrolysis of bacterial and microfaunal polysaccharides, as well as many secreted proteases, chitinases and glucanases, likely involved in the degradation of organic compounds in the litter. The absence of ligninolytic capacities points to a weak saprotrophic habit for L. bicolor . By contrast, these degradative functions are more limited in the truffle, making it intriguingly closer to animal-interacting fungi such as Malassezia globosa [14] , a yeast commonly found on the skin of many animals, including humans. Nutrient and signal exchange in EMs Mycorrhizal fungi, similar to other plant-interacting fungi, base their life cycle on the uptake of organic carbon from a living plant [2] ( Fig. 3 ). Fifteen genes encoding putative hexose transporters have been annotated in the L. bicolor genome and many of them are upregulated during symbiosis. However, the genome lacks genes encoding invertases, the enzymes that hydrolyse sucrose (the most abundant sugar in plant tissues) to glucose and fructose, suggesting that L. bicolor depends on the glucose released by its green host. In contrast, T. melanosporum possesses one invertase gene, indicating its potential capacity to access the plant sucrose pool, whereas other EM fungi, Amanita muscaria and Hebeloma cylindrosporum , also metabolize fructose. Interestingly, Ustilago maydis , a biotrophic pathogen causing smut disease on maize, possesses a sucrose transporter localized on the plasma membrane [16] that allows the fungus to directly acquire sucrose with no need for secreted invertases. Such a range of mechanisms to access plant sugars thus seems to mirror some of the differences in nutritional strategies between symbiotic and pathogenic fungi. 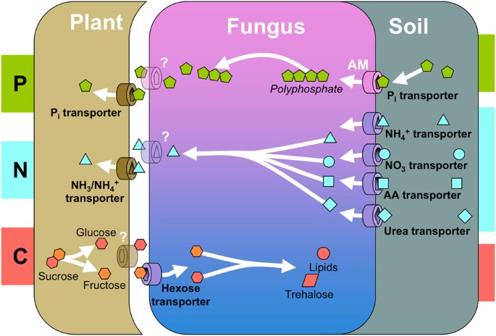Figure 3: Scheme summarizing the main nutrient exchange processes in EM and AM symbiosis. Emphasis is placed on the translocation of phosphorus (P), nitrogen (N) and carbon (C) at the soil–fungus and fungus–plant interface. Inorganic P and mineral or organic forms of N, such as NH4+, NO3−and amino acids (AA), are taken up by specialized transporters located on the fungal membrane in the extraradical mycelium. NH3/NH4+and Pi(the latter originated in AM fungi from the hydrolysis of polyphosphate) are imported from the symbiotic interface to the plant cells through selective transporters. Hexose transporters import plant-derived carbon to the fungus, whereas transporter proteins involved in the export of nutrients from either the plant or fungus have not been identified yet. This questions whether such processes indeed result from active, protein-mediated transport or involve passive export mechanisms. Figure 3: Scheme summarizing the main nutrient exchange processes in EM and AM symbiosis. Emphasis is placed on the translocation of phosphorus (P), nitrogen (N) and carbon (C) at the soil–fungus and fungus–plant interface. Inorganic P and mineral or organic forms of N, such as NH 4 + , NO 3 − and amino acids (AA), are taken up by specialized transporters located on the fungal membrane in the extraradical mycelium. NH 3 /NH 4 + and P i (the latter originated in AM fungi from the hydrolysis of polyphosphate) are imported from the symbiotic interface to the plant cells through selective transporters. Hexose transporters import plant-derived carbon to the fungus, whereas transporter proteins involved in the export of nutrients from either the plant or fungus have not been identified yet. This questions whether such processes indeed result from active, protein-mediated transport or involve passive export mechanisms. Full size image Mutualistic interactions are based on the exchange of nutrients; for this reason, genes coding for transporter proteins are expected to be well represented in EM fungal genomes. In spite of this prevision, the number of transporters annotated in L. bicolor is comparable to that of other saprotrophic and pathogenic fungi (491 genes), and they are even less abundant in T. melanosporum (381 sequences). However, many of these genes are upregulated in the symbiotic condition, implying very intense traffic of amino acids, oligopeptides and polyamines through the symbiotic interface [12] . Analysis of EM genomes highlights the capacity of the free-living mycelium to import organic and inorganic N sources, including nitrate, ammonium and peptides from the soil, through proteins such as the ammonium transporter or the urea permease ( Fig. 3 ). These functions are probably common to many EM fungi, as they were first described in A. muscaria ( AmAMT2 ) and Paxillus involutus ( PiDur3 ) [12] . From the mycelium, N compounds reach the mantle and the Hartig net, from where they can be exported to the plant; even if this mechanism is poorly understood, glutamine and ammonium are the best candidate molecules to cross the symbiotic interface [12] . This implies ammonium assimilation into amino acids and their translocation to the plant, or, alternatively, the direct release of ammonium ions from the Hartig net hyphae. A possible confirmation of the second alternative comes from the upregulation of ammonium importers in EM poplar roots [17] . Pathogenic fungi possess genes for a large array of secreted/effector proteins [18] . The discovery that L. bicolor possesses about 300 small cystein-rich secreted proteins that are upregulated during interaction with poplar and Douglas-fir opens new scenarios. For example, these proteins could function as effectors during the early phase of the plant–fungus interaction or could be involved in the construction of the symbiotic interface, as suggested by the immunodetection of one of these proteins (MISSP7) in the hyphal mantle [13] . These data point to the interface area as a site of recognition between the partners; however, comparable effector-like proteins have not been detected in T. melanosporum , leading to the question of whether EM Ascomycetes have developed alternative pathways for communicating with their hosts or whether such functions are carried out by other small secreted proteins. The wealth of information derived from the sequencing of L. bicolor , T. melanosporum and poplar [19] provides an opportunity to dissect the molecular basis of EM and unravel the regulatory networks that allow uptake, movement and exchange of nutrients between partners. However, plant transcriptomic responses are still limited, as only the poplar genes that respond to L. bicolor have been investigated [20] . Among the 39,303 genes on the poplar microarray, 2,945 were differentially expressed, including several transcripts encoding proteins involved in auxin metabolism and root morphogenesis. This finding has led to a model in which fungus-induced auxin accumulation at the root tip stimulates lateral root formation through auxin redistribution and auxin-based signalling. Sequencing the genomes of L. bicolor and T. melanosporum has therefore been a landmark in the study of fungal biology: the data illustrate similarities and differences among saprotrophic, symbiotic and pathogenic fungi and offer the first insights into the mechanisms behind fungal nutritional strategies. Genomic tools have transformed our understanding of the molecular mechanisms that regulate EMs, which may now become new models in plant–microbe interactions. Furthermore, they provide an appreciation of what makes a fungus a symbiont or a pathogen. Development of transformation protocols for EM fungi will permit the identification of molecular determinants that allow the transition from pathogenicity to saprotrophism or symbiosis, similar to that carried out for bacterial [21] and fungal species [22] in which few genes have been demonstrated to control the symbiotic status. AM fungi are the most widespread fungal symbionts of plants, being associated with more than 80% of current land plants [2] ( Fig. 1 ). They all belong to the phylum Glomeromycota, a monophyletic group that diverged from the same common ancestor as Ascomycota and Basidiomycota [23] . Although AM host plants can survive if deprived of their fungal symbionts, this condition is virtually unknown in natural ecosystems, in which AM fungi function as true helper microorganisms, improving overall plant fitness. Plants grown in artificial non-symbiotic conditions have shown that AM fungi significantly contribute to the uptake of soil nutrients, increase plant biomass and confer on the plant improved resistance to stress and pathogens [2] . In contrast, AM fungi have so far proved to be unculturable in the absence of a host. Being unable to absorb carbohydrates except from inside a plant cell, these fungi strictly depend on their green hosts for growth and reproduction, which gives them the status of obligate biotrophs. From an evolutionary point of view, the ecological success of AM fungi demonstrates that the advantages of such a strict association with plants have overcome the risks arising from the loss of saprotrophic capabilities. The unique biological features of AM fungi AM fungi are considered to be asexual, although the hyphae of genetically distinct strains can anastomose and exchange genetic material [24] , [25] . The very concepts of species and individual are poorly defined in this group of organisms, reflecting a high degree of genetic and functional variability. Even the definition of a cell as a hyphal compartment is inconsistent with the syncytial mycelia of these fungi, in which nuclei are constantly translocated by rapid cytoplasmic streaming [26] . Finally, their large asexual spores contain thousands of nuclei, making classical genetic approaches unsuitable [7] . A further level of complexity arises as several Glomeromycota host unculturable endobacteria. The meaning of this bacterial/fungal symbiosis has only recently begun to be investigated [27] , [28] , but the inability to culture both types of endobacteria, their vertical transmission and the small genome size of Candidatus Glomeribacter [27] strongly suggest that these endobacteria are ancient partners of AM fungi and may have been of evolutionary importance for fungal speciation [29] . All these unorthodox traits have so far limited the possibility of applying standard approaches such as genetic transformation, mutant generation and characterization, as well as large-scale transcriptomic and genomic analyses, to AM fungi. Although sequencing methods are evolving fast, the project to sequence the genome of the AM fungus Glomus intraradices has met a bumpy road [30] . Assembly difficulties for this relatively small genome (estimated to be around 14–16 Mb) are probably due to a high level of heterozygosity and/or to a larger genome than expected. At the same time, the lack of a uninucleate cell stage in the life cycle of AM fungi is a major obstacle in obtaining stable transgenic strains. Nevertheless, the transient expression of an exogenous gene in G. intraradices has been achieved through biolistic transformation [31] . Because of these peculiar traits, transcriptomic [32] and proteomic [33] analyses have so far proven to be more successful in investigating the molecular basis of AM fungal growth and function. In contrast to AM fungi, genetic tools and genomic information have helped in investigating several aspects of AM interactions such as root colonization and communication between symbionts [7] , [27] , [34] . Nevertheless, this one-way approach has very likely provided us with a biased picture, in which the plant seems to be the main factor and determining the contribution of each partner to the establishment and functioning of the association is still difficult. Understanding the functions of AM fungi The demonstration that AM fungi possess high-affinity inorganic phosphate (Pi) transporters provided a breakthrough in the understanding of fungal function. After the identification of a complementary DNA that encoded a transmembrane Pi transporter from G. versiforme , the function of the protein was confirmed by complementation of a yeast mutant affected in Pi transport [35] . Furthermore, the expression of this Pi transporter was localized to the extraradical hyphae of G. versiforme , the site of phosphate uptake from the soil ( Fig. 3 ). Accumulated as polyphosphate, Pi is then rapidly translocated along the aseptate mycelium to the host plant [36] . Nitrogen is another important element taken up by AM fungi, and genes involved in the transport of ammonium [37] and amino acids [38] have been identified, whereas arginine is probably the preferred molecule for long-distance transport to the host plant [39] . A glutamine synthase gene of G. intraradices is in fact preferentially expressed in extraradical hyphae, whereas a gene associated with arginine breakdown is expressed more in the intraradical mycelium. Although carbon transfer from plants to AM fungi was demonstrated in the 1960s [2] , its molecular mechanisms are still unclear. Surprisingly, with the exception of one gene from the non-AM Geosiphon pyriforme [40] , which hosts intracellular cyanobacteria, no hexose transporters responsible for C uptake from host cells have so far been characterized in Glomeromycota. The availability of expressed sequence tag libraries from different steps of the life cycle of G. intraradices will offer a more complete picture of fungal activity. A first glimpse has been caught by Seddas et al . [41] , who monitored G. intraradices genes involved in transcription, protein synthesis and metabolism in quiescent and germinating spores, as well as during interactions with wild-type and AM-defective (Myc − ) mutants of Medicago truncatula . The expression of only a few fungal genes is strongly affected by the plant genotype [41] . Although there are an increasing number of studies on specific fungal genes, the genetic traits that discriminate an AM fungus from an EM fungus or a pathogen are currently unknown. Interestingly, a G. intraradices gene , STE12-like , complements a non-invasive mutant of the pathogenic Colletotrichum lindemuthianum , restoring its infectivity [42] . Similarly, a gene encoding an Era-like GTPase in the rice pathogen Magnaporthe oryzae and required for virulence was found to be similar to the Gin-N protein from G. intraradices [43] . These findings suggest that some molecular mechanisms underlying the invasion of plant tissues are shared by pathogenic and symbiotic fungi, in spite of their distant phylogenetic relationships and diverse trophic habits. The dissection of plant responses illustrates how the mechanisms operating to accommodate the AM fungus inside the plant cell lumen are shared by diverse plants and have been conserved during evolution. Root colonization is vital to AM fungi ( Fig. 4 ). Their spores feed germinating hyphae through the catabolism of storage lipids for just a few days [2] . During this period, hyphae explore the soil in search of a host but if they never meet one, they arrest their growth and retract their cytoplasm back into the spore, which may again become dormant and restart the germination process over and over. This situation is not likely to be very frequent in nature because of the wide host range of these fungi, but is a hallmark of their obligate biotrophy, as well as their endurance. This strict biotrophy has long frustrated attempts to obtain enough material to perform large-scale nucleic acid extractions or produce sterile inoculum. The latter was made possible by root organ cultures that serve as a living substrate to grow several species of AM fungi [44] . 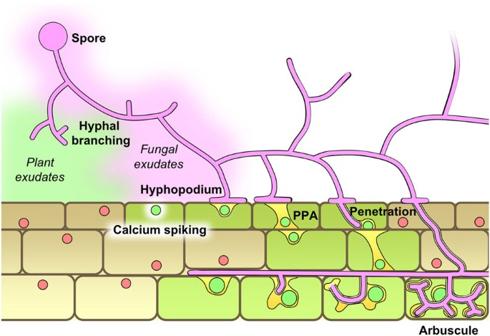Figure 4: Schematic summary of the root colonization process by AM fungi. The germination of a resting spore is followed by the production of a short explorative mycelium. The perception of plant exudates, released by the host root, induces recursive hyphal branching, increasing the probability of a direct contact between the symbionts. In the meantime, fungal exudates are perceived by the root, where they trigger calcium spiking through the activation of the common SYM pathway (Box 1). Signal transduction leads to the activation of cellular and transcriptional responses (green cells and nuclei). The contact between the plant and fungus is followed by the adhesion of a hyphopodium to the root surface. This triggers the assembly of a broad aggregation of cytoplasm (yellow), named the prepenetration apparatus (PPA) in the contacted epidermal cell and underlying outer cortical cell. Subsequent intracellular fungal colonization strictly follows the route of PPAs from the epidermis to the inner cortex. Here, intercellular hyphae can develop along the root axis. The PPA mechanism is then replicated in the contacted inner cortical cells, both before fungal entry and—on a smaller scale—branching. Eventually, a highly branched arbuscule occupies most of the cell volume, forming an extensive surface for nutrient exchange. Figure 4: Schematic summary of the root colonization process by AM fungi. The germination of a resting spore is followed by the production of a short explorative mycelium. The perception of plant exudates, released by the host root, induces recursive hyphal branching, increasing the probability of a direct contact between the symbionts. In the meantime, fungal exudates are perceived by the root, where they trigger calcium spiking through the activation of the common SYM pathway ( Box 1 ). Signal transduction leads to the activation of cellular and transcriptional responses (green cells and nuclei). The contact between the plant and fungus is followed by the adhesion of a hyphopodium to the root surface. This triggers the assembly of a broad aggregation of cytoplasm (yellow), named the prepenetration apparatus (PPA) in the contacted epidermal cell and underlying outer cortical cell. Subsequent intracellular fungal colonization strictly follows the route of PPAs from the epidermis to the inner cortex. Here, intercellular hyphae can develop along the root axis. The PPA mechanism is then replicated in the contacted inner cortical cells, both before fungal entry and—on a smaller scale—branching. Eventually, a highly branched arbuscule occupies most of the cell volume, forming an extensive surface for nutrient exchange. Full size image Strigolactones as a new class of bioactive molecules Perception of the host plant by the presymbiotic mycelium is mediated by root exudates. The responsible compounds that are released by the root and diffuse a short distance, before being washed away or degraded, have been identified as strigolactones [45] , [46] . They stimulate AM fungal metabolism and branching, a change in mycelial growth pattern that is thought to increase the chances of an encounter with the host. Strigolactones also have a hormonal role in inhibiting lateral branching of shoots [47] , [48] . This direct effect on plant development is considered to be the main function for this class of molecules, which are in fact produced by many plant taxa [45] , [49] , including those not associated with mycorrhizal fungi. The leakage of strigolactones from roots into the soil and their rapid hydrolysis have in any case made them ideal for signalling root proximity in the rhizosphere [7] , [49] . The seeds of parasitic weeds are also stimulated to germinate by strigolactones [50] . These multiple functions recall the pleiotropic effects of auxins, and promote consideration of strigolactones as hormones. The still uncharacterized Myc factors AM fungi are not inactive during their presymbiotic growth. A molecular dialogue precedes root colonization, keeping the partners informed about their reciprocal proximity [34] . Although the responsible molecules have not yet been identified, AM fungal bioactive molecules were shown to be smaller than 3 kDa, partially lipophilic [51] and suggested to possess a chitin backbone [34] . These diffusible signals, often referred to as 'Myc factor' [52] , are known to be perceived by the plant also in the absence of a physical contact with the fungus, inducing, for example, a membrane-steroid-binding protein, which is critical for mycorrhization [53] . Plant responses to Myc factors range from the molecular to the organ level and are part of a reprogramming under the control of the so-called common symbiosis (SYM) pathway ( Box 2 ), the signal-transduction pathway that prepares the plant for successful association with both AM fungi and nitrogen-fixing rhizobia. Box 2: The common symbiosis pathway Calcium spiking as a Rosetta stone for nodulation and AM The common SYM pathway seems to be primarily involved in controlling early events in AM establishment, and particularly the precontact responses and first steps of root colonization. Mutation of one of these genes blocks fungal colonization at the epidermal or subepidermal cell layer. The central factor of this signalling pathway is the most widespread second messenger in eukaryotic cells: the calcium ion. In addition to rapid calcium influxes, which are induced by both Nod factors [54] and AM fungal exudates [52] , the repeated oscillation of calcium concentration in the nuclear region of root hairs (Ca 2+ spiking) has long been observed in response to rhizobial signals [54] and used to position the activity of gene products along the SYM pathway. In recent years, specific calcium signatures have also been described for AMs. The proximity of branched hyphae was reported to induce Ca 2+ oscillations in the perinuclear cytoplasm of M. truncatula root hairs expressing the cytoplasmic calcium sensor Cameleon [55] . Although such cells are not usually infected by AM fungi, this observation represents the first evidence of an AM-induced Ca 2+ spiking response. The pattern of such Ca 2+ oscillations show several distinctive traits compared with those induced by nitrogen-fixing bacteria. The regular peak frequency that characterizes Nod factor-induced Ca 2+ spiking and the much more irregular pattern observed in AM responses have been modelled mathematically to suggest their chaotic nature [55] , [56] . These differences could be the key to understanding one of the central questions in the study of legume symbiosis: as the common pathway is shared by both AM and nodulation, how does the plant determine which microorganism is trying to colonize its tissues? This is anyway not the case for the majority of AM host plants, which have no obvious relationship with rhizobia. The search for Ca 2+ spiking responses to AM fungi in non-legumes therefore seems to be a promising field for providing insight into such mechanisms. Once a chemical acquaintance has been made between the fungus and the plant, and roots and hyphae have proliferated and branched in a small volume of the rhizosphere, the presymbiotic phase of the AM interaction culminates in a physical encounter between symbionts, when a hyphal tip touches the surface of a root ( Figs 4 and 5 ). AM fungi carefully select the location for starting root penetration. Hyphae can wander for several centimetres along the root surface, forming long, straight or gently curving hyphae; then, unpredictably, they swell, flatten on the cell wall of a few epidermal cells and branch repeatedly to develop what is known as a hyphopodium [57] . In the absence of direct evidence, several clues may shed light on this process. When the plant and fungus are separated by a permeable membrane, AM hyphal branching concentrates in the vicinity of young lateral roots [52] , which are also commonly acknowledged as the primary site of AM colonization, at least in laboratory conditions [58] . 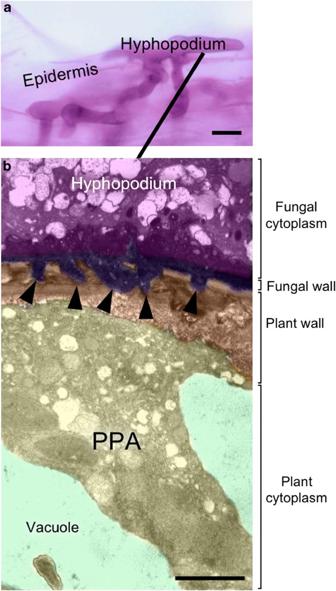Figure 5: Hyphopodium adhesion to the root epidermis in arbuscular mycorrhizas. A top view of the carrot root epidermis is shown ina, in which a branched hyphopodium ofGigaspora giganteastained with acidic fuchsin contacts the cell surface (bar, 10 μm). The transmission electron micrograph inbshows that the hyphopodium strict adhesion to the root is achieved through the formation of several protrusions of the fungal cell wall into the wall of the epidermal cell (arrows). A prepenetration apparatus (PPA), assembled in response to fungal contact, is visible underneath the hyphopodium as a broad column of cytoplasm traversing the vacuole (bar, 2 μm). Figure 5: Hyphopodium adhesion to the root epidermis in arbuscular mycorrhizas. A top view of the carrot root epidermis is shown in a , in which a branched hyphopodium of Gigaspora gigantea stained with acidic fuchsin contacts the cell surface (bar, 10 μm). The transmission electron micrograph in b shows that the hyphopodium strict adhesion to the root is achieved through the formation of several protrusions of the fungal cell wall into the wall of the epidermal cell (arrows). A prepenetration apparatus (PPA), assembled in response to fungal contact, is visible underneath the hyphopodium as a broad column of cytoplasm traversing the vacuole (bar, 2 μm). Full size image Hyphopodia tightly adhere to the root epidermis and their wall protrudes with many digitations into the outer layers of the plant cell wall ( Fig. 5 ). The molecular and developmental mechanisms mediating the switch from linear apical growth to the swollen and branched form of the hyphopodium are still completely obscure. By contrast, hyphopodium development is known to be followed by a pause in fungal growth that can last for 4–6 h before new tip growth is initiated to develop the penetration hypha [57] . During this time, plant cells and tissues prepare for colonization. The symbiotic pathway-dependent expression of ENOD11 (a gene coding for a putative secreted protein) is reported in the hyphopodium area [58] . The expression of several other plant genes also changes, many of which are already regulated during the presymbiotic phase [59] . New genes also become active on hyphopodium development, including those involved in cell wall remodelling and defence [60] , just at the time when epidermal cells reorganize their cytoplasm to produce an AM-specific structure that is indispensable for successful fungal penetration: the PPA (prepenetration apparatus) [57] . Contacted epidermal cells start to assemble the secretory machinery that builds the interface compartment where the fungus will be hosted. Cytoplasm becomes aggregated at the contact site, then develops into a thick column that predicts the subsequent route of the hypha across the cell [57] . All elements of the secretory pathway are concentrated in the PPA: abundant endoplasmic reticulum, and many Golgi bodies and secretory vesicles [61] . But the main factor in this display is the nucleus; at an early stage, its movements to and from the contact site anticipate PPA development [57] . Eventually, the PPA is completed and the fungus starts growing again, with a hyphal tip heading through the epidermal cell wall and along the track of the PPA. At this time, the perifungal membrane is thought to be assembled, as PPA secretory vesicles are expected to fuse to produce an invagination of the plant plasma membrane. Perifungal membrane development marks the appearance of the symbiotic interface, the narrow intracellular compartment that allows AM fungi to grow inside the plant cell without breaking its integrity [5] ( Figs 4 and 6 ). 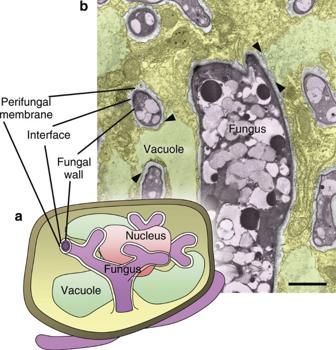Figure 6: The organization of an arbusculated cortical cell. The scheme inashows how intracellular fungal hyphae are enveloped by the perifungal membrane, an extension of the host cell plasma membrane. This outlines the interface compartment, an apoplastic space that surrounds the fungus and mediates nutrient exchange. The central vacuole is resized into a smaller volume as the fungus develops to occupy most of the cell lumen. The nucleus enlarges and is positioned in the middle of the hyphal branches. The transmission electron image inbshows the details of the fungal accommodation process inside an arbusculated cell of carrot. The interface compartment (uncoloured) is clearly visible all around the fungus (pink), whereas plant organelles are observed all around the perifungal membrane. In particular, the tonoplast occasionally seems to be in direct connection (arrows) with the perifungal membrane (bar, 2 μm). Figure 6: The organization of an arbusculated cortical cell. The scheme in a shows how intracellular fungal hyphae are enveloped by the perifungal membrane, an extension of the host cell plasma membrane. This outlines the interface compartment, an apoplastic space that surrounds the fungus and mediates nutrient exchange. The central vacuole is resized into a smaller volume as the fungus develops to occupy most of the cell lumen. The nucleus enlarges and is positioned in the middle of the hyphal branches. The transmission electron image in b shows the details of the fungal accommodation process inside an arbusculated cell of carrot. The interface compartment (uncoloured) is clearly visible all around the fungus (pink), whereas plant organelles are observed all around the perifungal membrane. In particular, the tonoplast occasionally seems to be in direct connection (arrows) with the perifungal membrane (bar, 2 μm). Full size image All AM fungi are characterized by—and named after—arbuscules (from the Latin arbusculum , small tree, Fig. 6 ). These structures are formed in the inner root cortex by repeated branching of an intracellular hypha, and considered the site of nutrient exchange [62] . The mechanisms controlling arbuscule development are largely unknown. The colonization step is not strictly dependent on the common symbiotic pathway, as, under high inoculum pressure, a few SYM mutants can be forced into AM colonization [63] . In most of these cases, the development of arbuscules proceeds normally, although their overall distribution is sometimes reported to be more limited and patchy [7] . Some genes that affect arbuscule development have been recently identified by reverse genetics. RNA interference knockdown of the Vapyrin gene, coding for a cytoplasmic protein with unknown function, induces a marked decrease in epidermal penetration and a total block of arbuscule formation [64] . In this case, only intercellular hyphae develop between cortical cells. This form of hyphal growth also spreads AM infection along the root in wild-type plants and is likely to be less strictly controlled by the plant, as it takes place outside the cells. Similarly, silencing of either a subtilisin protease [65] , a phosphate transporter [66] or two ABC transporters [67] results in arbuscular morphogenetical defects. Taken together, these findings suggest that genes essential for arbuscule development may be independent of the SYM signalling pathway. The fungal accommodation process Although the regulatory mechanisms leading to fungal branches filling most of the host cell lumen are poorly understood, the process of arbuscule accommodation, which requires a substantial remodelling of the cortical cell, has long been described [5] , [6] , [7] . Similar to any intracellular hypha, all the thin arbuscule branches are enveloped by the perifungal (now periarbuscular) membrane. This invagination of the host plasmalemma does not simply surround the arbuscule as a whole, but closely follows the surface of each branch, moulded to the arbuscule itself. The arbusculated cell is where the interface acquires its maximum spatial complexity, with a composition very similar to that of plant primary cell wall [5] . The assembly of this extensive amount of membrane and cell wall material requires the recursive involvement of PPA-like structures, organized both in advance of fungal penetration through the cell wall and along the 'trunk' hypha, as smaller aggregates anticipating the formation of fungal branches [61] . The periarbuscular interface assembly also involves the proliferation of endoplasmic reticulum, Golgi apparatus, trans -Golgi network and secretory vesicles [61] , [68] , as well as AM-induced subtilases secreted at the symbiotic interface [65] . This is not the only restructuring that the cortical cell undergoes. Plastids multiply and deploy around the fungus, interconnected by their stromules [69] . The nucleus and nucleolus increase in size, whereas chromatin is decondensed [61] , a likely mark of enhanced transcriptional activity. When first the PPA and later the arbuscule occupy a considerable part of the cell volume, the vacuole also has to be reorganized. Although a detailed in vivo analysis of tonoplast dynamics (and the mechanisms involved) is not yet available, it is clear from confocal microscopy that the vacuole is markedly reduced in size [68] , closely following hyphal branches ( Fig. 6 ). Arbuscules are ephemeral structures with an estimated lifespan of 4–5 days. At the end of this cycle, the fungal walls start to collapse in the arbuscule fine branches, as the cytoplasm retracts. Eventually, this process of senescence extends to the trunk hypha until the whole arbuscule is shrunk to a compact mass of hyphal cell walls. During this process, the periarbuscular membrane rearranges once more to adapt to its changing content. The fungus eventually disappears and the host cell regains its previous organization with a large central vacuole [70] and can undergo new colonization. In fact, root infection by AM fungi is not a linear or synchronous event. As the fungus repeatedly attempts cell (and root) colonization, arbuscules of very different ages coexist in neigbouring cells, and early structures, such as young hyphopodia, can develop on already colonized roots. How arbusculated cells operate The significant cell reorganization during root colonization is associated with important changes in the transcriptomic profile of AM roots. Several model plants have been investigated, including M. truncatula [71] , [72] , [73] , rice [74] and L. japonicus [75] , in which more than 500 protein-coding genes were found to be differentially regulated during the arbuscular phase. In all cases, expression level was significantly altered for genes, including those for nutrient transporters, transcription factors and proteins involved in cellular dynamics and cell wall synthesis. A mycorrhiza-specific plant phosphate transporter, which is localized on the periarbuscular membrane [6] ( Fig. 3 ), is essential for active symbiosis [66] . Among the regulated L. japonicus genes, 47 putative transporters were identified; 28 of them may be important for nutrient acquisition and are considered as novel markers for AM roots. The strongest upregulated gene of the array is a putative ammonium transporter [76] , the transcripts of which have been quantified and specifically localized in arbusculated cells using laser microdissection. The availability of microarrays and novel molecular tools has stimulated questions on the systemic effects of AM fungi [77] in plants of agronomic interest as well. Significant gene modulation was reported in shoots of mycorrhizal tomato [78] . The knockdown of sucrose synthase affects arbuscule development, and also reduces plant height, shoot weight and seed yield [79] . All these data support the idea that, on colonization, plants activate an organism-wide reprogramming of their major regulatory networks and argue that mobile factors of fungal or plant origin are involved in a generalized metabolic change; in this context, hormones [80] , [81] and microRNA [82] , [83] may be good candidates. At present, experimental data—for example, for jasmonic acid—are still highly controversial [80] , [81] . Analysis of ethylene, abscisic acid, salicylic acid and jasmonate-related compounds coupled to transcriptional profiling have documented both common and divergent responses of tomato roots to G. mosseae and G. intraradices [84] . The emerging picture looks complicated: symbiosis changes the levels of several hormones, in parallel with changes in the expression of their biosynthetic enzymes, also highlighting a role for oxylipins in AM [84] . Oxylipin regulation shows parallels with plant–pathogen interactions; as resistance to Phytophthora parasitica is known to depend partly on oxylipin synthesis in tobacco [85] , oxylipin regulation might shed light on the enhanced resistance of AM plants to pathogens [86] . In conclusion, the plant processes that permit the accommodation of fungal structures are active in epidermal, outer and inner cortical cells. They require orchestration among signal-transduction pathways, transcriptional and proteomic changes and major cell reorganization. Recent data clearly show that the long described 'growth effect' observed in AM plants depends on systemic consequences of the symbiosis, which go beyond the root system and affect the physiology of the whole plant. The idea that AM fungi have coevolved with plants since the past 400 million years, and that their association has helped the conquest of dry terrestrial ecosystems by Embryophyta [87] , is very popular. As lichens clearly show, combining an organism that can exploit light and atmospheric CO 2 with one that can efficiently exploit the substrate represents a fruitful adaptation to habitats at the soil–atmosphere interface. However, experimental data supporting the antiquity of AM associations have until recently been limited to fossils and the observation that extant AM fungi colonize basal plant lineages, including hepatics, hornworts and lycopods. The study of AM interactions in these plants can shed light on the origins of symbiosis, as they spend most of their life cycle haploid and do not possess roots [87] . AM fungi are known to colonize haploid gametophytic tissues with different degrees of success: whereas mosses such as Physcomitrella patens , a model basal plant, do not seem to undergo AM colonization, many hepatics and hornworts are successfully colonized both in the field [88] and in vitro [89] . The molecular biology of rootless plants and their interaction with AM fungi are poorly studied. However, recent findings [90] may represent a breakthrough: three SYM genes controlling symbiosis establishment in legumes [7] and monocots [91] have also been reported in basal plants ( Fig. 7 ), suggesting that AM colonization is a homologous process throughout Embryophyta, including both gametophytes and sporophytes. Furthermore, CCaMK orthologues from liverworts and hornworts can complement M. truncatula dmi3 non-mycorrhizal mutants. These results suggest that SYM genes were already present in ancestral plants and have been conserved during evolution. Finally, the finding of SYM genes in taxa that do not associate with AM fungi, such as Physcomitrella and Arabidopsis , could indicate that the corresponding proteins have likely been coopted to other functions, unrelated to AM symbiosis. 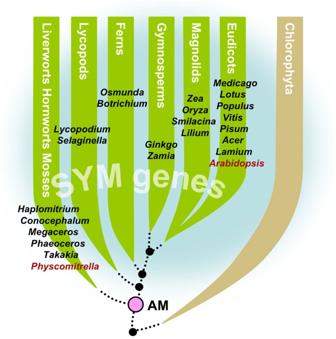Figure 7: The distribution of SYM genes in plant taxa. Phylogenetic and molecular evolutionary analyses91have demonstrated that the SYM genes controlling symbiosis establishment in legumes7and monocots90,91are distributed throughout Embryophyta, including both gametophytic and sporophytic phases of liverworts and other basal plants. By contrast, SYM homologues have not been detected in green algae (Chlorophyta), apparently relating the occurrence of SYM genes to terrestrial habitats. AM colonization can therefore be envisaged as a homologous process that was established by a common ancestor of all extant plant clades (pink node). Red colour highlights plant taxa that possess SYM gene homologues but do not establish AM. Figure 7: The distribution of SYM genes in plant taxa. Phylogenetic and molecular evolutionary analyses [91] have demonstrated that the SYM genes controlling symbiosis establishment in legumes [7] and monocots [90] , [91] are distributed throughout Embryophyta, including both gametophytic and sporophytic phases of liverworts and other basal plants. By contrast, SYM homologues have not been detected in green algae (Chlorophyta), apparently relating the occurrence of SYM genes to terrestrial habitats. AM colonization can therefore be envisaged as a homologous process that was established by a common ancestor of all extant plant clades (pink node). Red colour highlights plant taxa that possess SYM gene homologues but do not establish AM. Full size image When considering mycorrhizal symbioses in the context of current global challenges (environmental change, ecosystem conservation, sustainable agriculture, development of plants for future needs and food safety), we acknowledge that mycorrhizal fungi may be crucial in many of these fields: mycorrhizal fungi mobilize P and N, and are an important C sink in the soil, having therefore an important impact on the cycling of these elements [92] . As biofertilizers, they may counteract fertilization excess and thus promote sustainable agriculture. The selection of new crop varieties giving yields on poor soils and in low fertilization conditions should therefore consider new aspects, such as their responsiveness to mycorrhizal fungi, which has never consciously been taken into account during plant domestication [93] nor during modern breeding. Finally, food quality and security are strictly linked to the necessity of feeding a constantly growing global population under the threat of climate change; in this frame, unravelling the contribution of mycorrhizal fungi to the nutritional quality of edible plant organs becomes a priority. If the promises of mycorrhizal research are easy to catalogue, many constraints related to the biology of mycorrhizal fungi still limit their fulfilment. Identification of the signalling molecules released by AM and EM fungi is a first necessity. Although the potential Myc factor from AMs is currently under investigation [34] , on the basis of potential similarities with the Nod factor, the production of similar molecules did not emerge from the genomes of EM fungi; rather, there is evidence of the presence of small secreted proteins. Once this information is available, novel agricultural and forestal treatments can be envisaged, whereas the quest for the corresponding receptors in plants will begin. Another promising field is the study of microbes associated with mycorrhizal fungi and their role as a third component of symbiosis. Once these basic biological questions have answers, we will be ready to exploit the mycorrhizal fungal community hidden in the soil but quietly benefiting plants and humans. How to cite this article: Bonfante, P. & Genre, A. Mechanisms underlying beneficial plant–fungus interactions in mycorrhizal symbiosis. Nat. Commun. 1:48 doi: 10.1038/ncomms1046 (2010).